Reinforcement learning in professional basketball players Reinforcement learning in complex natural environments is a challenging task because the agent should generalize from the outcomes of actions taken in one state of the world to future actions in different states of the world. The extent to which human experts find the proper level of generalization is unclear. Here we show, using the sequences of field goal attempts made by professional basketball players, that the outcome of even a single field goal attempt has a considerable effect on the rate of subsequent 3 point shot attempts, in line with standard models of reinforcement learning. However, this change in behaviour is associated with negative correlations between the outcomes of successive field goal attempts. These results indicate that despite years of experience and high motivation, professional players overgeneralize from the outcomes of their most recent actions, which leads to decreased performance. According to rational choice theory, organisms make choices in order to maximize their well-being or utility. Reinforcement learning (RL) provides a theoretical framework to study how this goal can be achieved using past experience of actions and rewards [1] . The RL methods utilized by humans and animals have been a topic of intense research over the last decade. In these studies, a subject repeatedly chooses between several alternatives and is repeatedly rewarded according to its choices. Conducted in controlled laboratory settings, these studies have demonstrated that RL methods can account for some aspects of observed behaviour [2] . Importantly, in some of these studies neural activity was recorded, providing insights into the neural basis of decision making and learning [3] , [4] , [5] , [6] , [7] , [8] , [9] , [10] . Professional basketball provides a unique opportunity to characterize reinforcement learning in a repeated-choice setting by highly motivated human experts within their natural environment. In basketball, players are repeatedly required to make decisions in a complicated environment. The players are extremely motivated to make the right decisions and they undergo years of extensive training aimed at optimizing their decision-making processes. Field goal attempts (FGAs) are particularly instructive as the binary outcome of these decisions (made/missed) enables a quantitative analysis. Moreover, in basketball, made FGAs are rewarded by 2 or 3 points (pts), depending on the distance of the player from the basket. This allows us to separately study the timing of 2pt and 3pt shots, and examine how the ratio of 3pt to 2pt shots depends on the previous FGAs and their outcome. Finally, the decision to attempt a field goal seems fundamental to the success of the team and therefore the years of extensive training are expected to optimize this decision. By analysing sequences of FGAs, we found that the outcome of even a single FGA significantly affects a player's behaviour. In the framework of RL, this demonstrates that players update their policy on-line during the game, in accordance with their recent performance. However, such learning is not guaranteed to improve performance, unless it is derived from an accurate statistical model of the dynamics of the game. We show that in basketball this learning is associated with a decreased performance, manifested in decreased field goal percentage and decreased expected number of points. We hypothesize that despite their high motivation and extensive training, professional basketball players may overgeneralize from their very recent experience to their expected future performance. The effect of the outcome of an FGA on behaviour We examined the records of leading players from the National Basketball Association (NBA) and the Women's National Basketball Association (WNBA) in two regular seasons (see Methods) in order to assess how successes and failures in 3pt attempts affect players' choice behaviour. We compared the probability that a player's next FGA is a 3pt given that his/her previous FGA was a made 3pt to that probability given that his/her previous FGA was a missed 3pt. For example, we considered these conditional probabilities for the Most Valuable Player (MVP) of the 2007–2008 NBA season. We found that the outcome of a single 3pt had a substantial effect on his behaviour: the probability that he would attempt a 3pt following a made 3pt was 53% (77/144). It was substantially lower, 14% (34/245), after a missed 3pt ( P <10 −15 , two-tailed Fisher's exact test). A qualitatively similar effect was observed when analysing more than 200,000 FGAs of 291 leading NBA players: on average, the probability of attempting a 3pt after a made 3pt was significantly higher than that probability after a missed 3pt (0.41±0.01 versus 0.30±0.01; P <10 −7 , Monte Carlo permutation test, see Methods for details of population statistics). 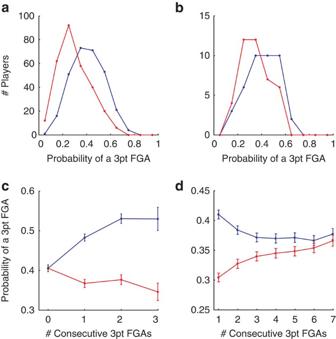Figure 1: The effect of the outcome of 3pt shots on players' policy. (a) Histograms of NBA players' probabilities of taking a 3pt shot following a made (blue)/missed (red) 3pt. (b) Histograms of WNBA players' probabilities of a 3pt shot following a made (blue)/missed (red) 3pt. (c) Probabilities of taking a 3pt shot conditioned on streaks of made (blue)/missed (red) 3pts. As some players did not have sufficiently long streaks of made/missed 3pts, this analysis was performed only on players who had streaks of three consecutive made 3pts and three consecutive missed 3pts; a total of 164 players. The difference between the red and the blue curves is significant (P<10−7, Monte Carlo permutation test) for all three points. The black dot at (0, 0.405) indicates that the average probability of attempting a 3pt across these players was 0.405. Error bars represent s.e.m. (d) Probabilities of a 3pt conditioned on a made (blue)/missed (red) 3ptn-FGAs ago,n=1,2, ... ,7. Error bars represent s.e.m. This is evident in Figure 1a where we plot the distribution over players of the probability of attempting a 3pt immediately after a made 3pt (blue) and after a missed 3pt (red). Note that the blue distribution is to the right of the red distribution. Interestingly, the sensitivity to the outcome of the previous 3pt shot, measured as the difference between the conditional probabilities, increased with the average number of minutes played per game ( r =0.18; P <0.01, t -test). Figure 1: The effect of the outcome of 3pt shots on players' policy. ( a ) Histograms of NBA players' probabilities of taking a 3pt shot following a made (blue)/missed (red) 3pt. ( b ) Histograms of WNBA players' probabilities of a 3pt shot following a made (blue)/missed (red) 3pt. ( c ) Probabilities of taking a 3pt shot conditioned on streaks of made (blue)/missed (red) 3pts. As some players did not have sufficiently long streaks of made/missed 3pts, this analysis was performed only on players who had streaks of three consecutive made 3pts and three consecutive missed 3pts; a total of 164 players. The difference between the red and the blue curves is significant ( P <10 −7 , Monte Carlo permutation test) for all three points. The black dot at (0, 0.405) indicates that the average probability of attempting a 3pt across these players was 0.405. Error bars represent s.e.m. ( d ) Probabilities of a 3pt conditioned on a made (blue)/missed (red) 3pt n -FGAs ago, n =1,2, ... ,7. Error bars represent s.e.m. Full size image The outcome of a single 3pt also had a substantial effect on the behaviour of women basketball players. Analysing more than 15,000 FGAs of 41 leading WNBA players, we found that the distribution of the probability of attempting a 3pt after a made 3pt (blue in Fig. 1b ) is to the right of that distribution after a missed 3pt (red in Fig. 1b ). On average, the probability of attempting a 3pt after a made/missed 3pt is 0.41±0.02/0.34±0.02 ( P <10 −6 , Monte Carlo permutation test). Because of the similarity in this effect between of NBA and WNBA players, their data were pooled together in what follows. In contrast to the significant effect of the outcome of 3pt shots on players' behaviour, successes and failures in 2pt attempts did not have a significant effect on the probability of the subsequent 3pt shot. The probability of attempting a 3pt after a made/missed 2pt is 0.344±0.007/0.340±0.007 (P >0.2, Monte Carlo permutation test). Therefore, we focused our analysis on the effect of 3pt shots on behaviour. The dynamics of learning In order to study the combined contribution of several events to choice behaviour, we computed the average probability of attempting a 3pt, conditioned on streaks of made 3pts (blue in Fig. 1c ) and missed 3pts (red in Fig. 1c ). These results indicate that the contribution of multiple successes and failures to behaviour is cumulative. Yet, players predominantly responded to the outcome of the last 3pt shot. To see this, we compared players' probability of attempting a 3pt shot following two consecutive 3pts with opposite outcomes. Given that the last two FGAs were a missed 3pt followed by a made 3pt, the probability of attempting a 3pt is 0.41±0.01. This number is significantly higher than that probability given that the previous two FGAs were a made 3pt followed by a missed 3pt, 0.33±0.01 ( P <10 −7 , Monte Carlo permutation test, 326 players). In order to find how long the outcome of a 3pt shot affects players' choice behaviour, we computed the probability of a 3pt shot, conditioned on a made/missed 3pt, n -FGAs ago, where n =1,2, ... ,7 (blue/red in Fig. 1d ). The difference between the red and blue curves indicate that the effect of a 3pt on behaviour diminishes within several FGAs (the difference between the two curves is significant for each of the first six points; P <0.05, Monte Carlo permutation test). In order to further quantify the dynamics of learning, we fitted the behaviour of the players to a RL model, in which the estimated values of the 2pt and 3pt shots are learned on-line (Methods). We allowed the model to have two different learning rates, η 2 and η 3 for the estimation of the values of the 2pt and 3pt shots, respectively, because the conditional-probability analysis indicated that the outcomes of 2pt and 3pt shots affect subsequent behavior differently. We used the method of maximum likelihood to fit the parameters of the model to the behaviour of each of the players (Methods). We found that despite substantial heterogeneity in the learning rates between the players, the sensitivity to the outcome of shots was predominant for the 3pt shots. This is reflected in the medians of the two learning rates in the population of players, η 2 =0.01 and η 3 =0.47. Moreover, qualitatively, the model captures the temporal dynamics of the 3pt probability of individual players ( Fig. 2 ). 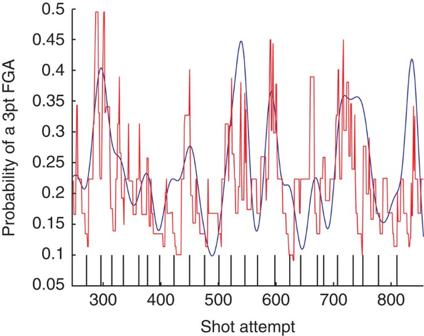Figure 2: A model of the learning behaviour of the MVP in 24 games in the 2007–2008 season. In blue, the empirical probability for a 3pt, computed by smoothing the attempted shots (a vector in which '1' indicated a 3pt attempt and '0' indicated a 2pt attempt) with a Gaussian filter whose s.d. was 10 FGAs. In red, the model prediction of 3pt probability as a function of FGA number, where numbers are counted from the beginning of the season. Black vertical lines indicate the beginning of a game. The similarity between the red and blue lines illustrates that the model captures some of the variation in the 3pt probability over time. Figure 2: A model of the learning behaviour of the MVP in 24 games in the 2007–2008 season. In blue, the empirical probability for a 3pt, computed by smoothing the attempted shots (a vector in which '1' indicated a 3pt attempt and '0' indicated a 2pt attempt) with a Gaussian filter whose s.d. was 10 FGAs. In red, the model prediction of 3pt probability as a function of FGA number, where numbers are counted from the beginning of the season. Black vertical lines indicate the beginning of a game. The similarity between the red and blue lines illustrates that the model captures some of the variation in the 3pt probability over time. Full size image Learning and performance are negatively correlated What is the effect of the change in behaviour on players' performance? Intuitively, increasing the frequency of attempting a 3pt after made 3pts and decreasing it after missed 3pts makes sense if a made/missed 3pts predicted a higher/lower 3pt percentage on the next 3pt attempt (3pt percentage is defined as the ratio between the number of made 3pts and the number of 3pts attempted). Surprizingly, our data show that the opposite is true. The 3pt percentage immediately after a made 3pt was 6% lower than after a missed 3pt (0.357±0.006 versus 0.378±0.006, P <0.01, Monte Carlo permutation test, 331 players). Moreover, the difference between 3pt percentages following a streak of made 3pts and a streak of missed 3pts increased with the length of the streak ( Fig. 3a ). These results indicate that the outcomes of consecutive 3pts are anticorrelated. 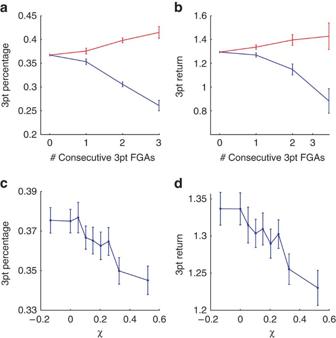Figure 3: Effect of learning on performance. (a) 3pt percentage following streaks of made (blue)/missed (red) 3pt shots. As some players did not have sufficiently long streaks of made/missed 3pts, the numbers of players considered were 331, 267 and 97 for 1,2 and 3 consecutive 3pt shots, respectively. Error bars represent s.e.m. (b) 3pt return conditioned on streaks of made (blue)/missed (red) 3pt shots. As ina, the numbers of players considered for the 1,2 and 3 consecutive 3pt were 331, 267 and 97 players, respectively. Error bars represent s.e.m. (c) Players were sorted into nine equal size groups according to their susceptibility (equation 1). For each group, the 3pt percentage is plotted as a function of the mean susceptibility. Error bars represent s.e.m. (d) Same sorting of players as inc; the 3pt return as a function of the mean susceptibility. Error bars represent s.e.m. Figure 3: Effect of learning on performance. ( a ) 3pt percentage following streaks of made (blue)/missed (red) 3pt shots. As some players did not have sufficiently long streaks of made/missed 3pts, the numbers of players considered were 331, 267 and 97 for 1,2 and 3 consecutive 3pt shots, respectively. Error bars represent s.e.m. ( b ) 3pt return conditioned on streaks of made (blue)/missed (red) 3pt shots. As in a , the numbers of players considered for the 1,2 and 3 consecutive 3pt were 331, 267 and 97 players, respectively. Error bars represent s.e.m. ( c ) Players were sorted into nine equal size groups according to their susceptibility (equation 1). For each group, the 3pt percentage is plotted as a function of the mean susceptibility. Error bars represent s.e.m. ( d ) Same sorting of players as in c ; the 3pt return as a function of the mean susceptibility. Error bars represent s.e.m. Full size image Increasing the frequency of attempting a 3pt after made 3pts and decreasing it after missed 3pts could also make sense if a made/missed 3pts predicted a higher/lower number of points earned by the team. In principle, it is possible that the decrease in 3pt percentage after a made 3pt is offset by other factors, such as an increased likelihood of getting the offensive rebound. In order to address this possibility, we considered the 3pt return, defined here as the average number of points gained by the offensive team from the time of the 3pt shot until the time that the opposing team got hold of the ball. Similar to the conditional 3pt percentage, the 3pt return immediately after a made 3pt was lower than after a missed 3pt (1.27±0.02 versus 1.34±0.02, P <0.01, Monte Carlo permutation test, 331 players). As was the case for 3pt percentage, the difference between 3pt returns following a streak of made 3pts and a streak of missed 3pts increased with the length of the streak ( Fig. 3b ). A change in the frequency of attempting a 3pt could have been justified if the outcome of 3pt shot was anticorrelated with the outcome of the following 2pt shot. However, there is no such effect: the 2pt percentage, following a made/missed 3pt was 0.460±0.005/0.468±0.004 ( P >0.16, Monte Carlo permutation test) and the 2pt return, following a made/missed 3pt was 1.20±0.01/1.22±0.01 ( P >0.08, Monte Carlo permutation test). Moreover, the changes in percentage and return that we observed were restricted to the shooting player: the 3pt percentage of other teammates immediately after a made/missed 3pt of a player was 0.366±0.009/0.349±0.006 ( P >0.11, Monte Carlo permutation test); the 3pt return of other teammates immediately after a made/missed 3pt of a player was 1.29±0.03/1.25±0.02 ( P >0.22, Monte Carlo permutation test). These results suggest that players attempt too many 3pt shots after a made 3pt, and too few after a missed 3pt. In order to further explore this possibility, we made use of the heterogeneity between players. We characterized each player according to the extent to which the outcome of a single 3pt attempt affects his/her 3pt probability. Formally, we define the susceptibility of a player, χ , to be the difference between the probability of a 3pt attempt following a made 3pt, Pr[3pt|made 3pt], and the probability of a 3pt attempt following a missed 3pt, Pr[3pt|missed 3pt] divided by the sum of these two probabilities: and characterize each player by his/her susceptibility. A positive susceptibility indicates that after a made 3pt, a player is more likely to attempt another 3pt, compared with after a missed 3pt. The larger the value of χ is, the stronger the effect of the outcome of a 3pt on a player's policy. We sorted the players into nine equal sized groups according to their susceptibility and computed the average 3pt percentage and average 3pt return for each group. The 3pt percentage ( Fig. 3c ) as well as the 3pt return ( Fig. 3d ) are negatively correlated with susceptibility, supporting the hypothesis that large positive susceptibility is detrimental to a player's performance. Learning is done by the shooting player We demonstrated that the probability at which players attempt 3pt shots depends on the outcome of their previous 3pt. We hypothesize that this results from a learning process taking place in the player's brain. Yet, there are other sources that could contribute to the observed change in behaviour. The change in 3pt probability could, in principle, originate from changes in the behaviour of players on the opposing team, as a result of learning processes taking place in their brains. However, this is unlikely because the defense is likely to try to prevent another 3pt attempt after a made 3pt and allow it after a missed 3pt. Such defensive manoeuvres are expected to decrease the magnitude of the observed learning. A change in behaviour of the player's coach or teammates could also contribute to the change in the rate of 3pts. For example, following a made 3pt, the coach may instruct the player to attempt more 3pts, or other teammates may pass more to the scoring player. While we cannot rule out these contributions, we found no evidence for this effect in the data. If the changes in a player's probability of attempting a 3pt are attributed to actions taken by the player's coach or teammates, we would expect the magnitude of the changes in different players on the same team to be correlated. For example, if the learning reflects the coach's instructions, we would expect similarity in the magnitude of learning of players on the same team, compared with players from different teams who are associated with different coaches. To test this hypothesis, we made use of the heterogeneity in the susceptibilities of the different players. We compared the within-team variance in susceptibility to the total variance by performing a one-way analysis of variance. The results of this analysis showed that the within-team variance in susceptibility was not significantly different from the between-teams variance in susceptibility ( P >0.53, one-way analysis of variance). Moreover, if changes in behaviour result from a learning process of the shooting player, susceptibility should be correlated over time. In order to test this prediction, we screened for players who passed our criteria in two seasons. For these players ( n =92), we compared susceptibility in the first season to the susceptibility in the second season. As predicted, susceptibility of players between seasons was positively correlated ( r =0.43, P <10 −4 , t -test). For comparison, the season-to-season 3pt percentage correlation coefficient for these players was 0.41. Taken together, these analyses suggest that the change in behaviour is at least partially due to processes taking place in the brains of the shooting players. The timing of FGAs is exponentially distributed So far we considered players' behaviour as a sequence of 2pt and 3pt attempts. In this framework, we quantified how past experience changes the probability that the next shot is a 3pt. This is reminiscent of standard two-alternative repeated-choice experiments, in which the course of the experiment is divided into discrete trials and a single binary decision is made on every trial [4] , [5] , [6] , [7] , [8] , [9] , [10] . However in basketball, the identity of the FGA, 2pt or 3pt is determined by the player's physical location. Therefore, at any particular point in time, a player does not choose between taking a 2pt and a 3pt shot. Rather, the player holding the ball chooses between attempting a field goal or not attempting one (for example, the player can move or pass the ball). In that sense, the game of basketball is more similar to free-operant procedures, in which animals choose between freely available alternatives [11] , [12] . To better understand the nature of decision making in basketball, we considered the timing of the FGAs of 204 NBA players for whom we could reliably determine this information (Methods). For each player, we computed the distribution of time durations between successive 2pt shots and between successive 3pt shots. We denote these durations as inter-2pt-intervals (I2Is) and inter-3pt-intervals (I3Is), respectively. 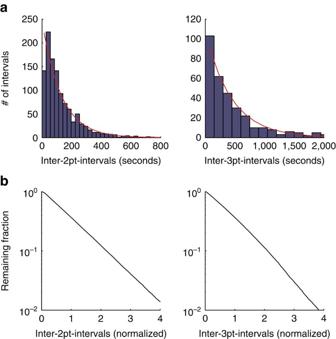Figure 4: Inter-FGA-intervals. (a) I2I (left) and I3I (right) histograms for MVP in the 2007–2008 season. Both histograms are well approximated by an exponential function (red line). (b) Normalized I2I (left) and I3I (right), averaged over the population of players, as a function of the fraction of intervals longer than an interval length ('survival plots'). Each player's I2Is and I3Is were normalized by the player's rates of 2pts and 3pts, defined as the number of 2pts/3pts attempts divided by the total duration of time played by the player. The normalized I2Is and I3Is were pooled together across all the players. The almost straight lines imply that the distributions of the I2Is and I3Is are well approximated by exponential functions (note the logarithmic scale of the ordinates). Histograms of MVP I2Is and I3Is in the 2007–2008 season appear in Figure 4a . The coefficients of variation (CV) of the I2Is and I3Is distributions are CV 2 =0.94 and CV 3 =1.08, respectively. These values are suggestive of an exponential distribution (for which CV=1). Indeed, both histograms are well approximated by an exponential function (red lines in Fig. 4a ). To further study the shape of the inter-shot-interval distributions, we considered the histograms of I2Is and I3Is of all players in our dataset. As the rates of FGAs of different players vary, we scaled the histograms of individual players by multiplying them by the rates of 2pt and 3pt shots, respectively, and averaged over all histograms (Methods). The normalized I2I and I3I distributions are depicted in Figure 4b (black lines) as 'survival plots': the fraction of intervals longer than an interval length, as a function of the length of the interval, for I2Is (left) and I3Is (right). In an exponential distribution, the fraction of intervals longer than a given interval decreases exponentially with the interval. Hence, the logarithm of the surviving fraction is a linearly decreasing function of the interval. The almost straight black lines in Figure 4b imply that similar to MVP's histograms, the distribution I2Is and I3Is in the population of players is also well approximated by an exponential function (note the logarithmic scale of the ordinates in 3B). Moreover, the CV for the population I2Is and I3Is distributions, CV 2 =0.93 and CV 3 =0.89, are also consistent with our observation that the distributions of I2Is and I3Is are approximately exponential. Figure 4: Inter-FGA-intervals. ( a ) I2I (left) and I3I (right) histograms for MVP in the 2007–2008 season. Both histograms are well approximated by an exponential function (red line). ( b ) Normalized I2I (left) and I3I (right), averaged over the population of players, as a function of the fraction of intervals longer than an interval length ('survival plots'). Each player's I2Is and I3Is were normalized by the player's rates of 2pts and 3pts, defined as the number of 2pts/3pts attempts divided by the total duration of time played by the player. The normalized I2Is and I3Is were pooled together across all the players. The almost straight lines imply that the distributions of the I2Is and I3Is are well approximated by exponential functions (note the logarithmic scale of the ordinates). Full size image Exponential distributions of inter-event-intervals are widespread in the natural sciences because they are the outcome of a homogeneous Poisson process, in which the probability of an event to occur at any point in time is constant and independent of previous events [13] . Thus, we explored the possibility that the timing of 2pt and 3pt shots can be approximated as resulting from two independent Poisson processes. In a Poisson process, the average time to the next event (waiting time) is independent of the initial time. Indeed, the average time from a 2pt to the next 3pt is comparable to the average I3I (351±7 and 352±6 s, respectively). Similarly, the average time from a 3pt to the next 2pt is comparable to the average I2I (211±5 and 209±4 s, respectively), consistent with the two independent Poisson processes description. Note, however, that the Poisson model is only an approximation. For example, we expect deviations from the Poisson model for very short and very long intervals: immediately following an FGA, the shooting player cannot attempt another shot. At the other extreme, the time until the next shot is bounded by the time to the end of the game. How does this Poisson-like behaviour emerge from the complex dynamics of a basketball game? In probability theory, it is well known that a Poisson process is a continuous time limit of a Bernoulli process, in which at any discrete time interval, a binary event occurs with some probability P . A Bernoulli process becomes a Poisson process in the limit of P →0 (denoting by Δ t the time interval, P =λ·Δ t and taking the limit Δ t →0 while keeping λ constant). Basketball is a dynamic game in which the ball is passed from one player to another every few seconds such that the temporal correlations in the state of the game are shorter than tens of seconds. If we partition the time line of the basketball game into contiguous slices that correspond to the correlation time of the game, we can consider each time slice as a Bernoulli trial in which the player takes an FGA with some probability P . Note that P <<1 because this correlation time is much shorter than the inter-FGA-interval, which is on the order of hundreds of seconds. Thus, Poisson-like behaviour emerges in basketball because the mixing time of the game is substantially shorter than the average inter-FGA-interval. Learning manifests as a change in rates If the timing of the 2pt and 3pt shots are generated by two Poisson processes, characterized by two rates λ 2 and λ 2 , respectively, then the probability that an FGA is a 3pt, P 3 , is given by . Therefore, in this Poisson framework, the learning described in the previous sections manifests as a change in the rates of the two processes. To study the effect of the outcome of a 3pt on λ 3 , we used the method of maximum likelihood to compute the average values of λ 3 triggered on the outcome of a 3pt. We found that on average, the value of λ 3 following a made 3pt was 2.83·10 −3 ±8·10 −5 sec −1 , 64% higher than its value after a missed 3pt, 1.73·10 −3 ±5·10 −5 sec −1 . Similarly, we computed the average values of λ 2 conditioned on the outcome of a 3pt. In comparison with the effect on λ 3 , the effect of the outcome of a 3pt on the value of λ 2 was modest: the average value of λ 2 triggered on a missed 3pt was 4.3·10 −3 ±1·10 −4 sec −1 , only 7% higher than its value after a made 3pt, 4.0·10 −3 ±1·10 −4 sec −1 . In this paper, we studied RL in professional basketball. We showed that players substantially change their behaviour, manifested as their rate of 3pt shots, in response to the outcome of a single 3pt. Moreover, this change is associated with decreased performance, as measured by 3pt percentage and 3pt return. These results provide insights into human RL in complex natural environments. The study of players' behaviour in professional basketball is not new. Previous studies, pioneered by Gilovich et al., [14] have already shown that players believe in the 'hot hand effect'; that is, they believe that following a streak of made/missed shots a player is more likely to make/miss a shot. Our contribution beyond previous studies is threefold. First, in previous studies, players' belief in the hot hand effect was revealed using questionnaires. In contrast, by considering the ratio of 3pt to 2pt shots and the distribution of inter-shot-intervals, we have shown that players' behaviour is consistent with such a belief. Second, we quantitatively characterized the dynamics of learning from experience in the game. Third, whether or not the outcome of successive FGAs is correlated has been debated for more than two decades [15] . We demonstrated that in the case of 3pt shots, in which players behaviour is substantially modified by their outcome, successive shots are negatively correlated. Intuitively, the decision of whether or not to attempt a field goal strongly influences the outcome of the possession. This assertion seems to contradict our empirical findings: despite the fact that on average, the rate of 3pts after a made 3pt was 64% higher than that rate after a missed 3pt, the difference in 3pt percentage and 3pt return between the two conditions was only 6%. This raises the question of why the outcome of a shot is so weakly dependent on the decision of when to make it. We hypothesize that this results from the strategic nature of the game. Consider a player holding the ball who contemplates taking an FGA or passing the ball. This decision can be made by estimating the expected payoffs from the two actions. For simplicity, we assume that the payoff is the return. At the same time, the players on the opposite team attempt to predict the player's decision in order to obstruct it. As the expected returns of the two actions, attempting a field goal or passing the ball, depend on the defensive manoeuvres, the player holding the ball attempts to predict the defensive manoeuvres. Previous studies have demonstrated that such interactions can lead to behaviours that follow a mixed Nash Equilibrium policy [16] , [17] , [18] . In a mixed Nash Equilibrium, the players choose their actions from a probability distribution, where the expected payoffs of all actions that are in the support of the Nash equilibrium is equal [19] . In this framework, the expected return from passing the ball and attempting the shot are equal. Let us now assume that as a result of a made 3pt, the player believes that attempting a shot is associated with a higher return than passing the ball. This would result in a significant change in his/her behaviour, shifting the policy from a random choice to attempting a shot. However, if the opposing team continues to play its Nash equilibrium policy (that is, they ignore the effect of the made shot on the shooting player's policy), there will be no change in the return of the shooting player because at the Nash equilibrium, the returns from all chosen alternatives are equal. In other words, in general, the decision to attempt a field goal is fundamental to the success of a player in the game. However, if all players choose their actions according to a mixed Nash equilibrium, the return in a shot will be independent of the chosen action (as long as it is in the support of the Nash equilibrium). We view the relatively weak dependence of the 3pt percentage on the rate of 3pts as indicative that the policies used by players in the game are near the Nash Equilibrium. Standard models of RL assert that when deciding between alternative actions, agents prefer the action associated with the highest value. In the process of learning, the values of the different actions at different states of the world are modified according to the outcomes of past actions (Methods). Consider a player who is holding the ball in a particular state of the game. After making an action, for example, attempting a field goal, and observing its outcome, which values should he/she update and by how much? Determining the proper level of generalization is a fundamental difficulty in this learning process. At one extreme, the player may conclude that he/she misestimated the value of attempting a 3pt from that particular configuration of the game, for example, the particular locations, postures and velocities of all players at the time of the FGA. On the other extreme, a player may generalize and conclude that the he/she misestimated the values of all 3pt attempts in all configurations of the game. The advantage of the former approach of limited generalization is that in a stationary environment, such learning can lead to an accurate representation of the values of the different actions in all game configurations [1] . However, the disadvantage is that learning is expected to be slow because of the large number of different configurations and actions. In contrast, the latter approach that generalizes from one state of the game to many states allows for fast learning, enabling the player to adapt to a changing environment. However, the player risks the possibility of overgeneralization. Similar considerations apply to the question of the optimal learning rate, which determines the tradeoff between the speed and accuracy of adaptation. Theoretical considerations suggest that in stationary environments, the speed of adaptation should decrease with experience [1] . However, such change in speed of adaptation has not been reported even in relatively long (400 trials) two-alternative repeated-choice laboratory experiments using the stationary two-armed bandit reward schedule [20] . To test for a change in the speed of adaptation of the basketball players, we checked whether the average susceptibility changes over time. We found no statistically significant difference in the susceptibilities computed for the first and second halves of the season (on average, χ =0.16±0.01 versus χ =0.15±0.01, P =0.19, Monte Carlo permutation test) or the susceptibilities between the first and second season for the 92 players who passed our criteria in two seasons (on average, χ =0.17±0.02 versus χ =0.15±0.02, P =0.15, Monte Carlo permutation test). Our analysis revealed that the outcome of a 3pt shot substantially affects the behaviour of the player in subsequent FGAs indicates that the player generalized from the state of the game associated with one shot to the state of the game associated with the subsequent shots. One way of implementing such a generalization is to scale up, by the same factor, the values of all 3pts from all states following a made 3pt, and scale down the values of these actions following a missed 3pts. However, applying algorithms that generalize from one state to other states are not guaranteed to improve performance [21] . Indeed, the decrease in 3pt percentage and return associated with an increase in 3pt probability and 3pt rate indicates that the change in players' behaviour following made and missed 3pts is not justified by the statistics of the game. Thus, we hypothesize that despite their extensive training, players may overgeneralize by means of an oversimplified on-line learning processes. The dataset The sequences of FGAs were obtained from the full play-by-play accounts of games played in the 2007–08 and 2008–09 NBA regular seasons ( Supplementary Data 1 and 2 , respectively, downloaded November 17th 2009), as they appear on the official NBA webpage http://www.nba.com , and from the 2008 and 2009 WNBA regular seasons ( Supplementary Data 3 and 4 , respectively, downloaded on March 22nd 2010), as they appear on the official WNBA webpage http://www.wnba.com . Sequences of FGAs for players with the same surname playing for the same team could not always be differentiated, and were therefore discarded. Moreover, we only considered players who made at least 100 2pt and 100 3pt shots in the season. Our data set was comprised of 291 NBA players with an average of 805 FGAs per player (min=219, max=2003 and std=380), 243 of these were 3pt shots (min=101, max=593 and std=103), and 41 WNBA players with an average of 416 FGAs per player (min=209, max=647 and std=110), 147 of these were 3pt shots (min=102, max=244 and std=36). Handling shooting fouls A shooting foul occurs when a player is fouled while attempting a shot. In NBA and WNBA statistics, these events are considered as FGAs only if the shot was made despite the foul. However, the shooting player typically cannot predict that the FGA will be associated with a shooting foul. Therefore, we considered all these events as FGAs and they constituted ∼ 8.2% of the FGAs analysed. In contrast, when reporting field goal percentages, we used the NBA and WNBA standard definition of considering only made fouled shot attempts. This is because the return associated with fouled missed attempts is substantially higher than that of non-fouled missed attempts, due to the free throws awarded to the fouled player. Computing returns The return of an FGA was computed by considering all points gained by the team of the shooting player from the time of the FGA until the opposing team got hold of the ball. To compute this number, we took into consideration FGAs, offensive fouls, turnovers and the end of quarters. Statistical procedures All statistical analyses were within-player: the numbers were computed separately for each player and then were averaged over the players, giving equal weight to each player in the average; averages reported are accompanied by the s.e.m. In some cases, the number could not be computed for a player and the player was omitted from the analysis. In those cases we report the number of players analysed. For example, only 164 players had at least one streak of three made 3pt shots followed by another FGA and at least one streak of three missed 3pt shots followed by another FGA. Therefore, only those 164 players are reported in Figure 1c . When computing the statistical significance of results averaged over a population of players, we performed the following Monte Carlo permutation test: independently for each player in each season, we computed the empirical distribution of FGAs and their outcome: number of made and missed 2pt and 3pt shots and the empirical distribution of 2pt and 3pt returns. When considering the effect of an FGA on subsequent behaviour, we replaced, for each player, the subsequent FGAs with FGAs drawn from the player's empirical distribution and averaged over all players. Similarly, when considering the effect of an FGA on the subsequent 2pt and 3pt percentages and return, we replaced the outcome of the subsequent 2pt/3pt with surrogate outcomes drawn from the player's 2pt/3pt percentages and return and averaged over all players. Each reported P -value indicates the number of times out of 10 7 repetitions of this procedure in which the difference in the averages obtained from surrogate data exceeded the difference in the averages for the original data. For the analysis of players' teammates, we considered all the teammates as if they were a single player and proceeded using the same procedure described above. Timing of FGAs The data set used for computing the I2Is, I3Is and the rates of 2pt and 3pt shots consisted of sequences of FGAs together with the specific time for each FGA obtained from the full play-by-play accounts of games played in the 2007–08 and 2008–09 NBA regular seasons, as they appear on the official NBA webpage http://www.nba.com . As before, sequences of FGAs for players with the same surname playing for the same team were discarded, and we only considered players who made at least 100 2pts and 100 3pts in the season. Moreover, games whose full play-by-play account contained mistakes were discarded from the data set. We detected several types of mistakes: misplaced entries, shot attempts by players who were supposed to be on the bench and inconsistencies between the time played by a player as derived from the full play-by-play and the time played as appears on the boxscore page that sums up the statistics of the game. A single mistake was sufficient to discard the whole game. The reduced data set, comprised of 101,458 FGAs made by 204 NBA players, still exhibits the effect of a single 3pt shot on behaviour: the probability of attempting a 3pt after made 3pt is much higher than after a missed 3pt (0.42±0.01 versus 0.30±0.01, P <10 −7 , Monte Carlo permutation test). When computing the times of FGAs of players we used the game time. Moreover, we only considered the times at which the player was actually playing (and did not take into account the time intervals during which the player was sitting on the bench). The I2I and I3I normalized distributions were constructed by normalizing each players' I2Is and I3Is by their rates of 2pts and 3pts, defined as the number of 2pts/3pts attempts divided by the total duration of time played by the player. These normalized I2Is and I3Is were pooled together to construct Figure 4b . Note that this analysis gives more weight to players that attempted more field goals. However, when computing the conditional rates, the rates were computed separately for each player and then averaged, giving equal weight to each player in the average. The Q-learning model In order to further quantify the dynamics of learning, we fitted the behaviour of the players using a one-state Q -learning model. According to this model, the player evaluates the values of 2pt and 3pt attempts, Q 2 and Q 3 , by computing the exponentially weighted averages of the outcomes of past attempts: where t is an index of the shot attempt, η 2 and η 3 are the 2pt and 3pt learning rates, respectively, R ( t ) is the return, that is, the number of points earned from the time of the attempt until the end of the possession, a ( t ) ∈ {2,3} is the type of shot attempt t and δ i , a ( t ) is the Kronecker delta such that δ i , a ( t )=1 if attempt t was type i and δ i , a ( t )=0 otherwise. The probability that the next attempt is a 3pt attempt is a softmax function of the difference in values with a bias term: where β is a measure of the stochasticity of the algorithm and b is a parameter. This model is a modification of standard on-policy Q -learning, where we allow for different learning rates for the two alternatives and we add a bias term. In order to fit the parameters of the model to the behaviour of each of the players, we assumed that the initial conditions of the model in each game, Q 2 (0) and Q 3 (0) are the average 2pt and 3pt returns in the season and the value of b was chosen such that at time t =0, Pr[3] is equal to the empirical fraction of 3pt shots in the season. The learning rates and the measure of stochasticity were estimated using the method of maximum likelihood. We found substantial heterogeneity in the resultant parameters between the players. The medians of the fitted values of these parameters across the population were: η 2 =0.01, η 3 =0.47, β =0.26 and b =−1.98. In order to demonstrate the ability of the model to capture the learning behaviour, we considered MVP's behaviour in the 2007–2008 season. The parameters that best characterize his behaviour in that season are η 2 =2.7·10 −7 , η 3 =0.27, β =1.02 and b =−1.28. Using equation. (2), we computed the trajectories of the values of 2pt and 3pt attempts, and using equation (3), the predicted probability of 3pt attempts. These probabilities are plotted in Figure 2 for 24 games taken from the middle of the season (red). In order to compare this prediction to the actual choices, we estimated the instantaneous probability of a 3pt attempt by convolving a Gaussian filter with the sequence of FGAs (a vector in which '1' indicated a 3pt attempt and '0' indicated a 2pt attempt; blue line). How to cite this article: Neiman, T. & Loewenstein, Y. Reinforcement learning in professional basketball players. Nat. Commun. 2:569 doi: 10.1038/ncomms1580 (2011).